Ultrafast vapourization dynamics of laser-activated polymeric microcapsules Precision control of vapourization, both in space and time, has many potential applications; however, the physical mechanisms underlying controlled boiling are not well understood. The reason is the combined microscopic length scales and ultrashort timescales associated with the initiation and subsequent dynamical behaviour of the vapour bubbles formed. Here we study the nanoseconds vapour bubble dynamics of laser-heated single oil-filled microcapsules using coupled optical and acoustic detection. Pulsed laser excitation leads to vapour formation and collapse, and a simple physical model captures the observed radial dynamics and resulting acoustic pressures. Continuous wave laser excitation leads to a sequence of vapourization/condensation cycles, the result of absorbing microcapsule fragments moving in and out of the laser beam. A model incorporating thermal diffusion from the capsule shell into the oil core and surrounding water reveals the mechanisms behind the onset of vapourization. Excellent agreement is observed between the modelled dynamics and experiment. The growth and subsequent collapse of cavitation bubbles near rigid surfaces produce strong mechanical forces that can create localized surface damage. Cavitation has been studied since the days of Lord Rayleigh [1] in a hydrodynamic setting, largely due to its destructive effects on submerged machinery, such as ship propellers. Our improved understanding of cavitation has resulted in a considerable reduction of deleterious effects and has also provided insight in the possibility to control the cavitation phenomenon [2] , [3] . While hydrodynamic cavitation is inherently chaotic due to pre-existing cavitation nuclei in the flow [4] , acoustic cavitation using high-intensity ultrasound provides a fine ability to trigger and direct released energies leading to myriad important applications, such as ultrasonic cleaning [5] , [6] and sonochemistry [7] , [8] . In medical therapy, much attention has been paid to high-intensity focused ultrasound surgery [9] and shockwave lithotripsy [10] , which use controlled cavitation for treatments such as kidney stone fragmentation. The use of stabilized microbubbles [11] , [12] provides many advantages by lowering the threshold for activation and, moreover, presenting a well-defined and localized nucleation point. Such precise control, both in space and time, helps to guide promising and often delicate therapies such as sonothrombolysis [13] , [14] , [15] , [16] and ultrasound-triggered molecular uptake (sonoporation) across the blood–brain barrier [17] , [18] . In addition, localized drug and gene delivery strategies based on such approaches dramatically reduce the payload and avoid the side effects of systemic administration. Another physical pathway for cavitation is through thermal excitation, leading to boiling, commonly termed vapourization. Precise control of localized vapourization is achieved when laser-induced cavitation bubbles [11] , [19] , [20] , [21] , [22] , [23] , [24] are formed in the tight focus of a nanosecond pulsed laser where the medium is locally superheated. A recent study achieved a lowering in activation threshold in laser-induced cavitation by using a new class of phase change agents based on liquid perfluorocarbon (PFC) droplets [25] . The sub-micron droplets have a low boiling point and are metastable at body temperature. When nanoparticle-based optical absorbers are dispersed in the PFC, localized heat deposition and phase conversion are triggered at low laser fluences. These cavitation events produced acoustic responses more intense than those from the classical thermoelastic expansion mechanism usually applied in photoacoustics [26] , [27] . While this optical absorber-mediated laser cavitation approach shows great potential in diagnostic and therapeutic applications, the precise physical mechanisms associated with vapourization have not been clarified until now owing to the short timescales of the vapour bubble dynamics and its complex interaction with the nanoconstructs. In this work, we study a different model system that also produces controlled laser-induced cavitation, namely a single micron-sized polymeric capsule with an absorbing dye in the capsule shell. Since the capsule contents and absorbers are spatially separated, such capsules are expected to be chemically more stable and more versatile in choice of both absorber and payload compared with the well-studied PFC droplets. Single capsules are excited by a pulsed laser and their response is monitored through combined ultrahigh-speed imaging and sensitive acoustic detection. From an energy balance between the heated capsule shell and the vapour bubble formed and coupled to its radial dynamics we find an excellent agreement with the experimental observations. Beyond the classical photoacoustic effect with the high-power pulsed laser, capsules also respond to continuous wave (CW) laser excitation by emitting a strong sustained signal, as long as the laser is on. The experiments are supported by a thermal model showing that the polymer heats up through dye absorption resulting in the melting of the capsule shell and release of the heated reservoir load into the superheated water, thus leading to instant vapourization. The experimental study and its subsequent modelling show that the prolonged response is a result of repeated vapourization/condensation cycles and a complex interaction of the laser and the dyed polymer fragments. Response to pulsed laser excitation A 3-μm oil-filled capsule with a Nile Red dye contained in its 600-nm thickness polymeric shell is illuminated with a 6-ns single laser pulse at a wavelength of 532 nm. The absorption, and subsequent heating, leads to localized vapourization. The ultrafast optical recording of the vapourization event simultaneous with the measurement of the acoustical response gives insight into the initiation and resulting dynamics of the bubble formed. 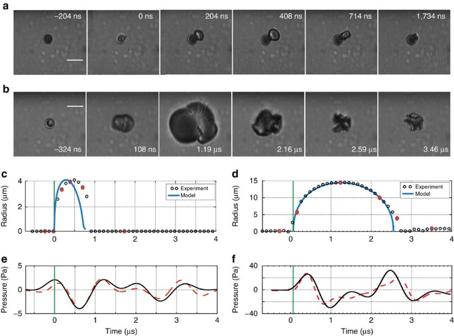Figure 1: Pulsed laser activation. (a) Still frames of the ultra high-speed recording of the growth and collapse of a vapour bubble with a laser fluence of 70 mJ cm−2(Supplementary Movie 1) and (b) of 1.4 J cm−2(Supplementary Movie 2). The scale bars represent 10 μm. (c,d) Radius–time curves of the events displayed ina,b; the filled circles correspond to the frames shown ina,b. The solid lines represent the proposed model (Equation (11)). (e,f) Pressure–time curves of the vapour bubbles froma,b. The dashed line represents the measurement, and the solid line represents the pressure computed from the radius–time curve and rescaled to the measured curve by a calibration factorA=0.7. A 60% reflection of the acoustic response from the microscope objective after 2.2 μs is included in the computed curves. Figure 1a,b shows a series of snapshots of the optical recording of the single oil-filled capsules excited by the laser pulse for laser fluences of 70 mJ cm −2 and 1.4 J cm −2 ( Supplementary Movie 1 and Supplementary Movie 2 ), respectively. When the laser light hits the capsule, the shell is disrupted while a bubble is formed that grows to a maximum radius of up to 15 μm in ~1 μs. After reaching its maximum radius, the bubble collapses, crumpling the polymer shell. Fluorescence emission, with a typical lifetime of a few nanoseconds, is too short to be detected within the 100-ns exposure time of the image recorded during the laser pulse. The radius–time curve was determined by tracking the contour of the bubble ( Fig. 1c,d ). Figure 1: Pulsed laser activation. ( a ) Still frames of the ultra high-speed recording of the growth and collapse of a vapour bubble with a laser fluence of 70 mJ cm −2 ( Supplementary Movie 1 ) and ( b ) of 1.4 J cm −2 ( Supplementary Movie 2 ). The scale bars represent 10 μm. ( c , d ) Radius–time curves of the events displayed in a , b ; the filled circles correspond to the frames shown in a , b . The solid lines represent the proposed model (Equation (11)). ( e , f ) Pressure–time curves of the vapour bubbles from a , b . The dashed line represents the measurement, and the solid line represents the pressure computed from the radius–time curve and rescaled to the measured curve by a calibration factor A =0.7. A 60% reflection of the acoustic response from the microscope objective after 2.2 μs is included in the computed curves. Full size image The acoustic pressure emitted by the bubble can be related to its radial oscillations [28] , [29] : where ρ w is the density of water, R the bubble radius, with and its time derivatives and r the recording distance. A is an empirical correction factor, equal to 0.7, and accounts for the far-field effect of the non-sphericity of the bubble oscillations, as well as the uncertainty in the transducer calibration. The acoustic signals measured simultaneous to the optical recording are shown in Fig. 1e,f , along with the calculated acoustic signals. The good temporal agreement suggests that the acoustic emission can be described by potential flow theory even in the present case of a vapourization event. In potential flow theory, the velocity field is described by the gradient of the velocity potential, a scalar function, and is applicable in inviscid irrotational flow, thus suggesting a negligible influence of vapourization and condensation on the overall system dynamics. The composition of the core of the microcapsules, oil or gas, did not significantly influence the overall response: the threshold for activation, the typical response signal frequency and the maximal bubble size were identical. The only difference was found after collapse, where minor rebounds were visible for the gas-filled capsules. The size and lifetime of the bubbles formed depend strongly on the applied laser energy. The activation threshold was found to be at a laser fluence as low as 70 mJ cm −2 . Such an energy level can easily be reached by a CW laser delivering typically 50 mW of power, focused in the same 10-μm-diameter focal spot for 1 μs. Therefore, we decided to investigate the response of both the gas- and oil-filled capsules when activated by a CW diode-pumped solid-state laser (5 Watt, λ =532 nm). 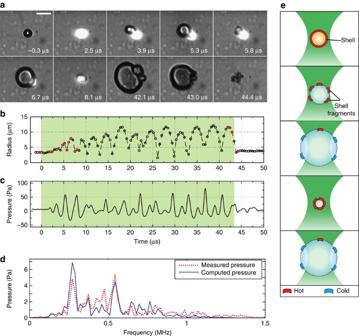Figure 2: Continuous wave laser activation. (a) Still frames from the ultra high-speed recording of a capsule irradiated by a continuous wave laser at 12 MW cm−2(Supplementary Movie 3). The scale bar represents 10 μm. (b) Radius–time curve of the bubble. Solid circles correspond to the frames ina. The shaded area represents the laser irradiation. (c) Measured acoustical response of the bubble ina. (d) Frequency content of the measured acoustic signal (dashed line). The solid line represents the frequency content of the calculated acoustic response. (e) Schematic representation of the vapour bubble formation and subsequent oscillations. The rod-shaped structures at the interface depict the absorbing polymer shell fragments resulting from shell break-up. They are pushed out of the laser focus during bubble growth, and the subsequent cooling leads to the collapse of the bubble, until the fragments return to the focus, where they heat up, and a new cycle is initiated. Response to CW laser excitation Figure 2 depicts the behaviour of an oil-filled capsule irradiated with a laser intensity of 12 MW cm −2 for a duration of 43 μs ( Supplementary Movie 3 ) and shows that CW laser illumination results in sustained oscillations of the vapour bubble. Here, as before, identical behaviour was observed for the gas-filled capsules and the oil-filled ones. During the first microseconds the capsule warms up while emitting a strong fluorescence signal. When the shell ruptures, a vapour bubble is formed, which grows and then continues to display stable oscillations. The oscillations can be explained by noting that the laser beam size is of the order of the capsule size. Figure 2: Continuous wave laser activation. ( a ) Still frames from the ultra high-speed recording of a capsule irradiated by a continuous wave laser at 12 MW cm −2 ( Supplementary Movie 3 ). The scale bar represents 10 μm. ( b ) Radius–time curve of the bubble. Solid circles correspond to the frames in a . The shaded area represents the laser irradiation. ( c ) Measured acoustical response of the bubble in a . ( d ) Frequency content of the measured acoustic signal (dashed line). The solid line represents the frequency content of the calculated acoustic response. ( e ) Schematic representation of the vapour bubble formation and subsequent oscillations. The rod-shaped structures at the interface depict the absorbing polymer shell fragments resulting from shell break-up. They are pushed out of the laser focus during bubble growth, and the subsequent cooling leads to the collapse of the bubble, until the fragments return to the focus, where they heat up, and a new cycle is initiated. Full size image Once the vapour bubble is formed, it expands beyond the resting radius defined by the thermal energy balance as a result of inertia. It can be seen in Fig. 2a that the fluorescent shell fragments follow the vapour/liquid interface and are therefore pushed out of the laser beam, where they cool down. This energy deficiency leads to condensation of the vapour bubble. The inertial collapse of the bubble leads to entrainment of the shell fragments back into the laser beam, leading to renewed absorption of energy for a new excitation cycle. This process is repeated while the fragments move in and out of the laser beam waist. When the laser is interrupted, the vapour bubble disappears instantly. The acoustic response of the microcapsule is shown in Fig. 2c and is calculated from Fig. 2a,b . The Fourier transforms of the measured and computed pressure signals are plotted in Fig. 2d . The signals contain a dominant frequency near 300 kHz and a pronounced harmonic component near 600 kHz. The threshold for the formation of a vapour bubble for CW laser excitation was found to be 1.0±0.2 MW cm −2 . Up to 12 MW cm −2 , the vapour bubble oscillations were not sustained for more than a few cycles, after which the vapour bubble stabilized at a resting radius balancing the absorbed and dissipated powers. Intensities above 12 MW cm −2 resulted in sustained oscillations of the vapour bubble during laser irradiation. Static thermal diffusion The process of heating up the polymer for the CW irradiation has to be treated in time. First, we determine the laser intensity required to heat up the polymer shell from its initial temperature T 0 to its melting point T melt (145 °C) [30] by solving the static thermal diffusion equation: with I being the laser intensity, R e and R i being the external and internal radii of the shell and λ p and λ w being the thermal conductivities of the polymer and the water, respectively. μ abs is the absorption coefficient of the dyed polymer and q e is the quantum yield of the dye in the polymer matrix. We performed experiments on Nile Red-doped polymer films with the same concentrations as those of the capsule shell with thickness of 50 μm and found a thermal conversion coefficient μ th = μ abs (1− q e )=43 cm −1 , corresponding to the fraction of absorbed light converted into thermal energy [31] . With the above μ th , we find from Equation (2) that the polymer melts at a laser intensity of 0.9 MW cm −2 , which corresponds very well with the experimental threshold for vapour bubble formation of 1 MW cm −2 reported above. Thus, it is very likely that the melting of the polymer triggers the vapourization event. Dynamic thermal diffusion Let us now solve the dynamic thermal diffusion equation and calculate the temperature profile within the shell as a function of time. We therefore use the substitution leading to the following equation for all three media: with P the density of thermal power, c p the specific heat capacity, ρ the density and D the thermal diffusivity. The boundary condition at the interface between the media 1 and 2 located at R is: where λ refers to the thermal conductivity. The system was solved using a finite element model, see the Methods section. All numerical calculations were performed in Matlab. Temperature evolution Details of the temperature evolution are displayed in Fig. 3 . A considerable temperature gradient develops within the capsule shell leading to a hot spot inside the polymer. The polymer thus melts in a localized zone within the polymer, while the shell melts gradually extending inward and outward with progressive laser heating and increasing temperature. Rupture of the polymer shell will occur when the thickness of the remaining solid polymer is of the order of the smallest defect in the shell, which was estimated to be near 4% of the wall thickness [32] . The location where rupture occurs is defined as the rupture point. Moreover, the presence of a solid and a melted phase in the shell requires the inclusion of the latent heat of fusion to correctly resolve the details of the temperature profiles. 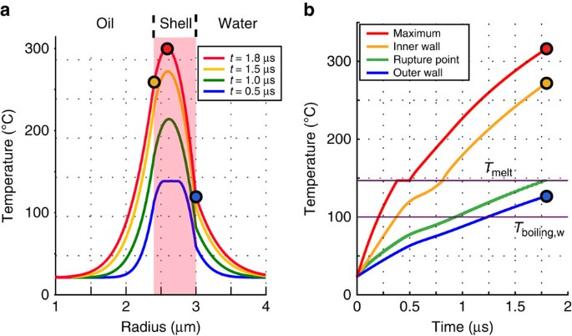Figure 3: Spatial and temporal temperature profiles. (a) Temperature profiles in and around the capsule during laser irradiation at four different time instants (laser starts att=0 μs). (b) Maximum temperature inside the polymer shell (red line) and at the inner wall (yellow line) and outer wall (blue line) of the shell as a function of time. Att=1.8 μs the temperature at the rupture point has reached the melting temperature,Tmelt=145 °C, while the oil has a temperature near 270 °C and the water at the outer wall is superheated above its boiling point at a temperature of 130 °C. Figure 3: Spatial and temporal temperature profiles. ( a ) Temperature profiles in and around the capsule during laser irradiation at four different time instants (laser starts at t =0 μs). ( b ) Maximum temperature inside the polymer shell (red line) and at the inner wall (yellow line) and outer wall (blue line) of the shell as a function of time. At t =1.8 μs the temperature at the rupture point has reached the melting temperature, T melt =145 °C, while the oil has a temperature near 270 °C and the water at the outer wall is superheated above its boiling point at a temperature of 130 °C. Full size image Four temporal snapshots of the computed temperature profiles are plotted in Fig. 3a . The temperature rise in and on either side of the polymer shell is plotted in Fig. 3b up to the time instant when the melting front reaches the critical rupture point. The model shows rapid heating of the polymer shell with higher temperatures at the inner wall due to similar thermal conductivities of oil and polymer compared with those of the polymer and water. Between t =350 ns and t =500 ns, the maximum temperature of the polymer gets pinned, as the phase change consumes part of the deposited heat and less is available for heat flow to the rest of the polymer, oil and water. At t =800 ns the shell is fully melted on the inner side, with the same pinning behaviour. Figure 3b also shows the temperature increase at the rupture point. Now the underlying physical mechanism of vapourization becomes apparent. Upon reaching the polymer melting temperature of 145 °C, the water has reached a temperature of 130 °C, thus slightly superheated around the particle, which does not lead to boiling in the absence of nucleation sites. The temperature at the inner wall is more than 100 °C higher, and upon reaching complete polymer melting, the heated oil flows into the superheated water leading to an instant vapourization of the water. Vapour bubble dynamics We now continue to describe the evolution of the vapour bubble, which we model by balancing the energy transferred from the polymer shell to the vapour bubble (which consists exclusively of water vapour) with the thermal losses at the vapour bubble interface. We assume that no light absorption takes place in the oil or water. No oil vapourizes since its boiling temperature is 286 °C. The shell is modelled by a rectangular slab of polymer with the same thickness and volume as the capsule shell, thereby conserving the diffusion time and total energy of the original problem. We write T e the temperature of the polymer slab following excitation. The temperature profile inside the polymer is calculated as a function of time using Fourier series, assuming a constant temperature T vap in the medium surrounding the slab. The temperature gradient at the walls leads to the power transferred from the polymer, and an integration over time results in the time-resolved energy transferred to the water W p : with where S p is the surface area of the wall and l is the wall thickness. The energy of a heated sphere of radius R when submerged in a water bath at room temperature is diffused towards the water across its thermal boundary layer δ that obeys the relation: where D w is the thermal diffusivity of water. The timescales of the experiment indicate that the temporal term is much larger than the spatial term 1/ R , which will therefore be neglected. To take in account the variation of the vapour temperature within the bubble due to the changes in pressure, we define an effective thickness δ R for the boundary layer that compensates for the subsequent variations in heat transfer from the vapour to the water. The new thermal boundary layer is therefore defined as: where T vap is the vapour temperature and T 0 is the ambient temperature. This definition cancels the temperature gradient for significant variations of the vapour temperature and is equivalent to the first one (Equation (5)) for small temperature variations. The existence of a temperature gradient results in the diffusion of thermal energy, giving rise to an energy loss W 1 from the vapour into the liquid: with λ w the thermal conductivity of water. We now describe the dynamics of the vapour/liquid interface using the Rayleigh–Plesset equation [4] , [28] : where P gas is the gas pressure, σ the surface tension of water, μ the viscosity of water, P 0 the ambient pressure and ρ w the density of water. The pressure is related to the energy (Equations (5) and (9)) through the gas law and enthalpy. Combining the three equations results in the following set of equations: where h vap is the vapourization enthalpy of water, c p,w the specific heat capacity of water and R g the gas constant. We accounted for the diverse damping elements of the system by increasing the theoretical liquid viscosity. The damping was measured from the decay of the free-field bubble oscillations following activation of the gas-filled capsules. The model predicts an initial temperature of the shell material far above the melting point of the polymer when high laser fluences are applied, as expected, thereby explaining the explosive-like growth of the bubble. At laser fluences just above the activation threshold, the polymer will be homogeneously heated in nanoseconds. At the moment of shell rupture, the inner polymer wall and adjacent gas or oil, and the outer polymer wall and adjacent water, will have been heated to the same temperature in excess of the melting point of the polymer (145 °C). Then, the same principle for the onset of vapourization is anticipated as was detailed for the CW irradiation: rupture of the shell leads to mixing of the heated inner core fluid into the superheated water to finally cross the potential energy barrier for vapourization. This matches the observations of small cavitation bubbles emerging from a single spot on the capsule shell ( Fig. 1a ). A direct comparison of the model (Equation (11)) and the experimentally obtained radius–time curves is plotted in Fig. 1c,d , where we indeed find excellent agreement. The results show that the biocompatible polymeric microcapsules can serve as absorbers for laser-induced cavitation, localized both in space and time, and which respond to both pulsed and CW laser irradiation. The physical modelling of the vapourization process is in excellent agreement with the experimental observations and shows the threshold step-control offered by the system. The dye encapsulation offers easy tuning of the absorption wavelength of the agent. The homogeneous bulk nucleation temperature of water is known to be higher than the temperatures considered here. The required energy rise to cross the potential barrier for phase conversion was attributed to the flow of preheated oil into the superheated water. In the case of microcapsules with a gas core, the surrounding water also undergoes vapourization upon rupture, with the difference that the existing gas pocket acts as a nucleation site by itself with a size larger than the critical nucleus radius [35] , thereby initiating the vapourization process. The absence of any sign of cavitation for dyed polymer solid spheres under similar laser illumination conditions demonstrate the importance of the presence of a liquid or a gas core. The design of the capsules allows for the encapsulation of a payload in the core, making them versatile agents for triggered release of drugs or genes. In this preliminary design, the capsules are already activated at powers close to those applied in the medical range, making them potentially powerful contrast agents for combined drug delivery and photoacoustic imaging [26] . For the suggested application of the CW laser, the sustained oscillations are a result of the motion of the vapour bubble in and out of the laser beam. The frequency of these oscillations will be governed by the Rayleigh–Plesset-type dynamics of a gas microbubble (Equation (11)) with a resting radius and initial bubble wall velocity that is directly coupled to the laser intensity and spot size. Thus, changing the laser spot size while maintaining an incident laser intensity above the threshold will change the frequency of the oscillations, which can be monitored acoustically. The CW laser, in principle, restricts the acoustic emission to the case of a single capsule. Nevertheless, a high-frequency modulation of the laser intensity would have a similar effect on the activation of the capsules without the strong focusing requirement and this will open up a wealth of promising opportunities for novel CW photoacoustic modalities. For medical imaging and therapeutic applications, it is important that the capsules are of a size around 100–200 nm to permit extravasation from leaky tumour vasculature. We are investigating synthesis aspects to downsize the capsules. It is expected that the production processes are closely similar, barring a few differences in the dynamics of capsule formation. It is also expected that similar levels of dye incorporation can be attained as in the larger entities. The mechanisms developed in this work will be applicable to the smaller capsules, and only for ultrasmall structures below the critical nucleation sizes will the model require a major overhaul. We are also investigating methods to lower the laser-induced cavitation threshold to ensure that the applied laser fluence stays below the maximum permissible exposures for human tissue. One approach is to use absorbers such as plasmonic nanoparticles with a larger absorption cross-section than typical dyes [36] . Another promising approach is to use a core of a low boiling point liquid, such as perfluorocarbons, encapsulated in a polymer shell with a low melting temperature [37] . Such a system would not be limited by the high boiling point of water and could present a more stable response in diverse environments. An approach to further reduce the cavitation threshold without modifications to the capsule is to synchronize laser light application with the creation of localized low pressures aided by focused ultrasound [38] . Microcapsules Two types of capsules were studied, both displaying identical behaviour: gas-filled capsules containing nitrogen and oil-filled capsules filled with hexadecane (see Fig. 4 ). The capsules had a narrow size distribution with a mean radius of 3.0±0.3 μm. Both microcapsules had fluorescent Nile Red dye incorporated in their shells as displayed in Fig. 4c,d , which shows the confocal fluorescence image of a gas-filled capsule and the oil-filled form, respectively. Absorption spectroscopy showed that the maximum absorption of the dye-doped shell was at 530 nm, which coincides with the frequency-doubled Nd:YAG laser emission. 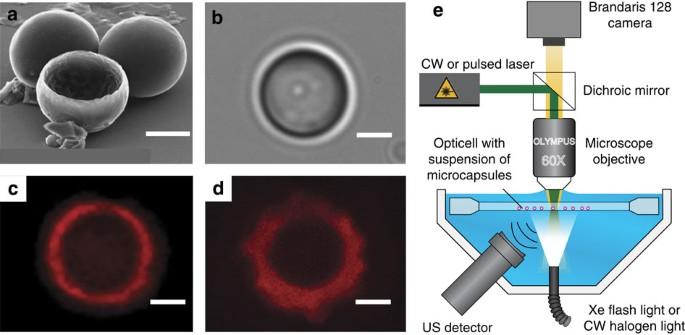Figure 4: Microcapsules and experimental setup. (a) Scanning electron microscopy image of hollow polymeric microcapsule, scale bar represents 5 μm. (b) Bright field and (c) confocal fluorescence image showing the distribution of dye within an oil-filled capsule and (d) that of a gas-filled capsule. The scale bars represent 2 μm. (e) Schematic representation of the combined optical and acoustical setup. The laser beam is focused through a × 60 objective on a single capsule placed in an Opticell. Ultrahigh-speed movies were recorded with the Brandaris 128 camera at 2–15 million frames per second. Figure 4: Microcapsules and experimental setup. ( a ) Scanning electron microscopy image of hollow polymeric microcapsule, scale bar represents 5 μm. ( b ) Bright field and ( c ) confocal fluorescence image showing the distribution of dye within an oil-filled capsule and ( d ) that of a gas-filled capsule. The scale bars represent 2 μm. ( e ) Schematic representation of the combined optical and acoustical setup. The laser beam is focused through a × 60 objective on a single capsule placed in an Opticell. Ultrahigh-speed movies were recorded with the Brandaris 128 camera at 2–15 million frames per second. Full size image The microcapsules were produced using ink-jet printing technology as described by Böhmer et al. [30] . The emulsification and subsequent lyophilization process allow for a well-controlled capsule size and shell thickness (see Fig. 4a,b ). The shell of the capsules consists of poly-L-lactic acid with a fluorinated hydrophobic end group of perfluorooctanol [39] , [40] . The Nile Red dye was incorporated into the shell material at a concentration of 0.1 wt% to make the polymeric capsules fluorescent without affecting the polymeric physical properties. Experimental setup The combined optical and acoustical behaviour of the capsules was studied by introducing a diluted suspension of the microcapsules into an Opticell container placed in a water bath ( Fig. 4e ). The chamber is optically and acoustically transparent. The laser light was focused on the sample in a 10-μm-diameter spot through a water-immersion objective ((LUMPLFL, × 60, NA=0.9, Olympus). The Brandaris 128 ultrahigh-speed camera [41] , [42] was used to make optical recordings (128 images; FOV of 80 × 60 μm) through the very same objective at frame rates ranging from 2 to 15 million frames per second. A sufficient illumination was reached by using a Xenon flash light. The acoustic signals emitted by the cavitation events were recorded at the bottom of the water bath by a 1-MHz focused broadband transducer (C302, Panametrics), then fed into a pre-amplifier (5077PR, Panametrics) and stored using a digital oscilloscope (DPO3034, Tektronix). The optical focus and the acoustic focus were co-aligned using a 0.2-mm-diameter needle hydrophone (Precision Acoustics, UK). A frequency-doubled Nd:YAG pulsed laser (Nano-PIV, Litron Lasers) was used for pulsed excitation (pulse width Δ t =7 ns, λ =532 nm) and a CW diode-pumped solid-state laser (5 Watt, λ =532 nm, Cohlibri, Lightline) was used for CW excitation as well as fluorescence imaging. The CW laser output was gated in time between 1 and 50 μs by an acousto-optic modulator (AOTF.nC-VIS, AA Optoelectronic) and its amplitude was controlled by the internal power settings. Analysis The radius–time curves were derived from the measured area taken from an automated bubble contour detection. As the capsule or polymer fragments cannot be distinguished from the vapour in the grayscale image frames, the following segmentation analysis was applied to separate out three distinct temporal regions. The first region is before laser exposure and corresponds to the capsule free of vapour. The second region is during the coexistence of the capsule/polymer fragments and the vapour. The third region results from the detection of the polymer fragments after complete collapse of the vapour bubble. The first and third regions can be distinguished within the optical recording as shown in Fig. 1a,b and are therefore easily corrected. In the second region, for the lower energy case ( Fig. 1a ) the measured bubble size can be corrected for by subtracting the capsule area from the total detected surface area. For the higher energies, with the complete melting of the capsules and explosive vapour bubble growth, the contribution of the polymer fragments leads to a negligible increase in the total surface area, and is therefore not taken into account. Numerical models The model presented in Fig. 1c,d was computed using the Matlab ODE45 and ODE113 solvers to solve Equation (11). In order to compute the theoretical acoustic emission of the vapour bubbles, the measured radius was interpolated numerically using a spline method and was filtered in the Fourier domain. This operation filters the measured noise with a significance similar to the natural filtering effect of the transducer bandwidth. The resulting curve was used as an input to Equation (1). Experimentally, a significant acoustic signal is received from the reflection on the microscope objective as can be observed in Fig. 1e . The reflection coefficient amounts to a value of 60±5% and a fixed delay of 2.2±0.2 μs; therefore, it could be included in the computed pressure–time curve. This issue becomes more complex in the case of the CW laser irradiation and can be avoided by comparing the signals in the frequency domain (see Fig 2d ). The finite element model was elaborated from the spherical heat diffusion equation (Equation (3)). The physical system formed by the capsule, the oil and the surrounding water obeys the following set of equations: with the substitution , as before. In the equations, the subscript p refers to the polymer, w to the water and oil to the oil. P represents the density of thermal power, c p,p the specific heat capacity of the polymer, and D and λ are the thermal diffusivity and the thermal conductivity of the materials, respectively. R i and R e represent the inner and the outer radius of the capsule, respectively. A fixed step finite element mesh was chosen (3 nm) and the Galerkin method is used to rewrite the previous system of equations on the basis of finite elements in order to conserve the influence of the second derivative in space. The system is discretized in time using a finite difference as the equations make use of only the first derivative in time. In the above equations, δ t is the time step and δ r is the spatial step used in the computation. The brackets refer to a vector and the double overbars refer to a matrix. [ a k ] is the amplitude vector of the function within the finite element functions array. [ δ k ] is the vector representation in finite element form of the heat creation term. The matrices and represent the decomposition of the term and on the finite element basis, respectively, and have a size that depends on the resolution of the computational grid. The boundary conditions are differentiated with respect to time to allow rewriting in the form of a single matrix system and implying the continuity of temperature: where is an invertible matrix that includes the boundary conditions: with the identity matrix. Table 1 lists the material properties used in the simulation. The stability of the model requires a simulation time step δ t of 0.01 ns. The boundaries of the simulation are taken at a distance of 6 μm from the centre of the capsule, where the effect of heat diffusion is negligible, at a constant temperature equal to the ambient temperature. During the computation, the latent heat of fusion of the polymer is taken into account by storing the energy created at each point ( dE = c p,p ( T − T melt )) in a temporary variable and adapting the temperature of the concerned points to the melting temperature ( T = T melt ) until the temporary variable reaches the required enthalpy of fusion. Table 1 Thermal material properties used in the finite element model. Full size table How to cite this article: Lajoinie, G. et al. Ultrafast vapourization dynamics of laser-activated polymeric microcapsules. Nat. Commun. 5:3671 doi: 10.1038/ncomms4671 (2014).